Global heat and salt transports by eddy movement Oceanic mesoscale eddies contribute important horizontal heat and salt transports on a global scale. Here we show that eddy transports are mainly due to individual eddy movements. Theoretical and observational analyses indicate that cyclonic and anticyclonic eddies move westwards, and they also move polewards and equatorwards, respectively, owing to the β of Earth’s rotation. Temperature and salinity (T/S) anomalies inside individual eddies tend to move with eddies because of advective trapping of interior water parcels, so eddy movement causes heat and salt transports. Satellite altimeter sea surface height anomaly data are used to track individual eddies, and vertical profiles from co-located Argo floats are used to calculate T/S anomalies. The estimated meridional heat transport by eddy movement is similar in magnitude and spatial structure to previously published eddy covariance estimates from models, and the eddy heat and salt transports both are a sizeable fraction of their respective total transports. Estimates of eddy heat transport are conventionally made in an Eulerian framework. Three approaches have been used: the first is the direct calculation of the covariance between temperature and velocity anomalies, , in the intraseasonal frequency spectrum band [1] , [2] , [3] ; the second is the assumption that the covariance is associated with geostrophic turbulent dispersion and is equal to the mean temperature gradient ∇ times an eddy diffusion coefficient, which itself must be independently estimated [4] ; and the third is the calculation of the V ′ T ′ product based on the vertical phase shift between temperature and geostrophic velocity associated with baroclinic instability [5] , [6] , [7] . None of these methods explicitly identify eddy movement, which is more naturally considered in a Lagrangian framework. Theoretical and observational analyses indicate that cyclonic and anticyclonic eddies usually move westwards, and they also move polewards and equatorwards, respectively, because of the β of Earth’s rotation [8] , [9] . T/S anomalies inside individual eddies (with respect to the ambient water) occur due to geostrophic uplift and depression of the background pycnocline vertical profiles associated with cyclonic and anticyclonic eddies, respectively. The sign of the T/S anomaly tends to be opposite in cyclonic eddies from anticyclonic eddies. The T/S anomalies tend to move with the eddies owing to advective trapping of interior water parcels, so eddy movement causes heat and salt transport. If information is available about eddy location and movement, and the associated T/S anomalies, then eddy heat and salt transport can be estimated by assuming that the compensating currents outside the eddies do not have correlated T/S anomalies on average. Automated eddy detection schemes have been applied to data sets from different surface observations [9] , [10] , [11] . They can be combined with the accumulating data sets on T/S vertical profiles from Argo profiling floats to directly estimate the heat and salt transport due to eddy movement. Using an eddy data set from satellite altimeter sea surface height anomaly (SSHA) data and T/S profiles from Argo floats, this study shows that the westwards zonal transport of heat and salt by cyclonic and anticyclonic eddies offsets each other, but they enhance each other in the meridional direction. The estimated meridional heat transport by eddy movement is similar in magnitude and spatial structure to previous eddy covariance estimates from models [1] , [2] , and the eddy heat and salt transport each is a sizeable fraction of its respective total transport [3] , [12] . The demonstrated importance of eddy transport supports the need for eddy-resolving oceanic models in climate simulations. Detected eddies and co-located Argo profiles A velocity geometry-based automated eddy detection scheme [13] is applied to surface geostrophic velocity anomalies derived from SSHA data to detect sea surface eddies. The Archiving, Validation and Interpretation of Satellite Oceanographic data (AVISO) multiple satellite-merged SSHA product is used, which has a spatial resolution of 1/3° × 1/3° and a 7-day temporal sampling over a period from January 1993 to December 2010 (Dong et al. [14] ). The detected eddy data set carries the information of eddy centre location, time, eddy polarity, eddy size, eddy boundary curve and eddy movement velocity. A global eddy data set is derived from the AVISO data using this method; it is available online [15] . Eddy statistical and dynamical characteristics in the subtropic frontal zone of the Northern Pacific Ocean were previously analysed based on this eddy data set [10] . The T/S vertical profiles of Argo floats from August 1999 to December 2010 are used [16] , and the T/S data are linearly interpolated onto 100 evenly spaced depth levels from 10 to 1,000 m. Individual profiles of T/S anomalies, T ′( z ) and S ′( z ), are calculated by subtracting the average over all Argo profiles within 5° × 5° bins. Given the large number of Argo profiles now available, the time-mean profiles are comparable to the Levitus climatological data [17] . All T/S profiles available within a detected eddy boundary around a specified date are collected and their anomalies are averaged. As the SSHA data are composited every 7 days, Argo T/S profiles within a 3-day interval of the composite time are treated as if simultaneous with the composite SSHA. The spatial distribution of the number of Argo vertical profiles within eddies in 5° × 5° bins is shown in Fig. 1 . In the North Pacific Ocean, for example, 7,249 and 8,131 Argo profiles are located inside cyclonic and anticyclonic eddies, respectively, out of a total of 203,904 Argo profiles. On the other hand, 6,531 and 7,141 cyclonic and anticyclonic eddies contain at least one Argo vertical profile, which indicates that few eddies have multiple profiles. However, most bins contain multiple eddies, especially in the Northern Hemisphere. An example of the T/S anomaly vertical profiles in the bin at [35°N–40°N] × [160°E–165°E] is shown in Fig. 2 . 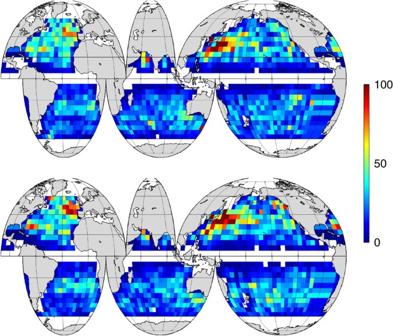Figure 1: Argo profiles trapped by eddies. The spatial distribution of the number of Argo profiles within cyclonic eddies (upper panel) and anticyclonic eddies (lower panel). The bin size is 5° × 5°. Figure 1: Argo profiles trapped by eddies. The spatial distribution of the number of Argo profiles within cyclonic eddies (upper panel) and anticyclonic eddies (lower panel). The bin size is 5° × 5°. 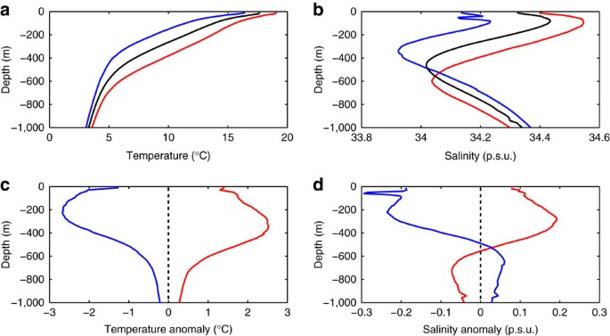Figure 2: Vertical profiles of T/S affected by eddies. An example of bin-averaged T/S vertical profiles from Argo data in the bin located at [35°N–40°N] × [160°E–165°E]: temperature (a), salinity (b), temperature anomaly (c) and salinity anomaly (d). Blue and red lines are for cyclonic and anticyclonic eddies, respectively, and the black lines are the means from all profiles. Full size image Figure 2: Vertical profiles of T/S affected by eddies. An example of bin-averaged T/S vertical profiles from Argo data in the bin located at [35°N–40°N] × [160°E–165°E]: temperature ( a ), salinity ( b ), temperature anomaly ( c ) and salinity anomaly ( d ). Blue and red lines are for cyclonic and anticyclonic eddies, respectively, and the black lines are the means from all profiles. Full size image Heat and freshwater transports by eddy movement We assume the eddies move coherently as bulk entities at all levels. For a single eddy with radial size r e , horizontal movement velocity , and T/S anomaly profiles , the horizontal heat and salt transports Q e are calculated by with units of W for heat and kg s −1 for salt mass, respectively. ρ o =1,025 kg m −3 and C po =4,200 J kg −1 °C −1 are mean upper-ocean density and heat capacity. The vertical integral is calculated by discrete summation over the interpolated vertical levels. The size of an eddy varies vertically. Modelling and observational experience has shown that there are three types of oceanic eddies in terms of vertical shape [18] : bowl, lens and cone shaped. Most eddies are bowl shaped. The coefficient s is set to 0.5 as a conservative choice of the vertical shape effect on eddy flux; that is, this is the minimum prefactor in equation (1), associated with a cone. Within each bin we average all the eddies that have simultaneous movement and T/S profile measurements (denoted by angle brackets). As only a fraction of the SSHA-detected eddies also have Argo profiles, we estimate the total time-mean transports by eddy movement by multiplying the average single eddy by the detected population number density N e within each bin, where N e is the total detected eddy number multiplied by the sampling interval of altimetry data (7 days) and divided by the time length of the analysis period; that is, The salt mass transport can be reinterpreted as an equivalent freshwater volume transport assuming conservation of mass across the transport section; that is, F fw =− T s / ρ o S o , where S o =35 p.s.u. (salt mass fraction) is the mean upper-ocean salinity. The unit of F fw is m 3 s −1 . Section-integrated, time-averaged heat and salt mass transport by cyclonic and anticyclonic eddy movement in the North Pacific Ocean are shown in Fig. 3 . In the zonal direction, because of the differing cyclonic and anticyclonic eddy movement and pycnocline displacement tendencies, both eddy types have negative zonal velocity (westwards propagation), so zonal heat and salt mass transport by the two types of eddies have opposite sign and tend to offset each other; hence, the total zonal eddy transport is generally smaller than by either type of eddy alone. In the meridional direction, however, where both the eddy propagation velocity and the heat and salt anomalies usually have opposite sign, the heat and salt transports by the two types of eddies have the same sign and mostly combine to give larger values than from either type alone ( Fig. 3 ). The spatial structure of the transport estimates is noticeably non-smooth on the 5° spatial resolution scale, suggestive of a degree of undersampling because too few eddies are detected. Mesoscale eddy fluxes have severe sampling errors, especially for conventional covariance-based estimates [19] . 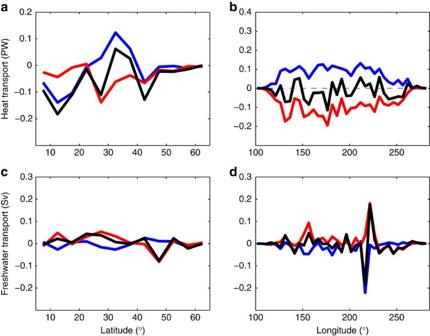Figure 3: Heat and freshwater transports by eddy movement in northern Pacific Ocean. Section-integrated, time-averaged heatQh(a,b) and saltQs(c,d) transports by eddy movement in the North Pacific Ocean. Panelsaandcand panelsbanddare for the shore-to-shore zonally integrated meridional (northwards) and [7.5–62.5°N] meridionally integrated zonal (eastwards) transport components, respectively. The blue, red and black lines are for the cyclonic, anticyclonic and total transports, respectively. Figure 3: Heat and freshwater transports by eddy movement in northern Pacific Ocean. Section-integrated, time-averaged heat Q h ( a , b ) and salt Q s ( c , d ) transports by eddy movement in the North Pacific Ocean. Panels a and c and panels b and d are for the shore-to-shore zonally integrated meridional (northwards) and [7.5–62.5°N] meridionally integrated zonal (eastwards) transport components, respectively. The blue, red and black lines are for the cyclonic, anticyclonic and total transports, respectively. Full size image Taking a global view, the zonally integrated meridional heat transport by eddy movements is plotted in Fig. 4 . No estimate of transport by eddy movements is made within [5°S–5°N] owing to a problematic geostrophic approximation near the equator. We superimpose two previous estimates [1] , [2] based on the first conventional approach defined above (anomaly covariance) using oceanic model simulations. All three results are similar both in the magnitude of the eddy heat transport, several times 0.1 PW (10 15 W), and in the general distribution with latitude. The discrepancies among these estimates are from uncertainties associated with each one. The estimation uncertainty in the current estimate depends on the spatial and temporal sampling frequency of vertical profiles of T/S within detected oceanic eddies (see Methods). 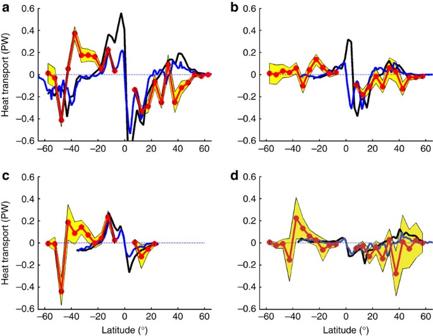Figure 4: Comparison with model results for eddy-induced heat transport. Comparison of zonally integrated, time-averaged meridional heat transports by eddy movementQh[PW] in red with Jayne and Marotzke1in black, and Volkovet al.2, in blue: World Ocean (a), Pacific Ocean (b), Indian Ocean (c) and Atlantic Ocean (d). The uncertainty range of the eddy heat transport by the eddy movement is indicated by the yellow shading. The data from Jayne and Marotzke1are digitized from their paper, and Volkovet al.2provided their data to the authors. Figure 4: Comparison with model results for eddy-induced heat transport. Comparison of zonally integrated, time-averaged meridional heat transports by eddy movement Q h [PW] in red with Jayne and Marotzke [1] in black, and Volkov et al. [2] , in blue: World Ocean ( a ), Pacific Ocean ( b ), Indian Ocean ( c ) and Atlantic Ocean ( d ). The uncertainty range of the eddy heat transport by the eddy movement is indicated by the yellow shading. The data from Jayne and Marotzke [1] are digitized from their paper, and Volkov et al. [2] provided their data to the authors. Full size image The primary structure is a heat transport convergence in the tropical zone and divergence in the subtropical and subpolar zones; that is, eddies transport heat towards the equator in the tropical zone in both hemispheres. This structure is evident in all three oceanic basins, but it is the clearest in their global combination. Its magnitude is a sizeable fraction (about 20–30%) of the total meridional heat flux in the tropical ocean but in the opposite direction [12] . A polewards transport is also indicated in the Southern Ocean. While the different estimates disagree by tens of percent in particular bins, they are remarkably consistent on the larger scale. This agreement implies, in particular, that eddy movement is a primary, if not dominant, mechanism for eddy heat transport. The global-scale estimate of salt transport by eddy movement is shown in Fig. 5 , expressed in terms of the equivalent freshwater volume flux F fw [Sv]. The overall magnitude is several times 0.1 Sv. The meridional transport patterns are approximately equatorial divergence, near-equatorial convergence and extratropical divergence, albeit with considerable variation on the bin scale. This magnitude is a moderate fraction (about 20–30%) of the ~1 Sv of the total oceanic meridional freshwater transport. The eddy flux pattern is congruent with the total flux pattern of freshening the evaporative subtropical zone and depleting the precipitative equatorial and extratropical zones [12] . An application of the second conventional estimation approach (with an eddy diffusivity) to the observed ∇ yielded an estimate [4] nearly an order of magnitude larger than the present eddy movement estimate and, therefore, is somewhat implausible. The estimated eddy freshwater flux has the same order of magnitude as that from an eddy-resolving model in the Southern Hemisphere [3] , and it has similar latitudinal variation with northwards flux in the middle latitudes; however, the present estimate exhibits more variability with latitude. Thus, we conclude, albeit with somewhat less confidence than for heat transport, that the contribution of eddy movement to salt transport also seems likely to be significant. 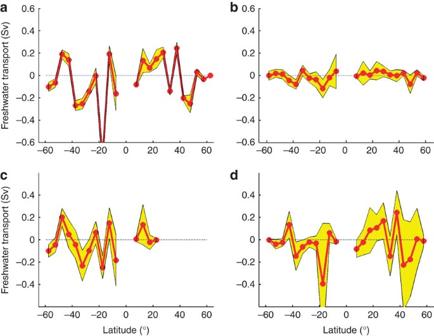Figure 5: Freshwater transport by eddy movement. Zonally integrated, time-mean freshwater meridional volume transport Ffw[m3s−1] by eddy movements, converted from the salt mass transportQsby multiplication by −1/(ρ0S0): World Ocean (a), Pacific Ocean (b), Indian Ocean (c) and Atlantic Ocean (d). The uncertainty range of the eddy heat transport by the eddy movement is indicated by the yellow shading. Figure 5: Freshwater transport by eddy movement. Zonally integrated, time-mean freshwater meridional volume transport F fw [m 3 s −1 ] by eddy movements, converted from the salt mass transport Q s by multiplication by −1/( ρ 0 S 0 ): World Ocean ( a ), Pacific Ocean ( b ), Indian Ocean ( c ) and Atlantic Ocean ( d ). The uncertainty range of the eddy heat transport by the eddy movement is indicated by the yellow shading. Full size image Uncertainties associated with the present eddy flux estimate are primarily due to the paucity of the observational data. Despite the sizeable number of Argo profiles available, only those trapped in eddies are useful for our analysis. Owing to the lack of full spatial and temporal coverage of eddies by Argo profiles, we had to use bin averaging and then zonal or meridional averaging to obtain the results shown in Figs 3 , 4 , 5 . The s.e. arising from such averaging (that is, the s.d. of all independent samples divided by the square root of the number of samples) are less than 0.1 PW for eddy heat flux and less than 0.1 Sv for freshwater flux. It should be noted that the point-to-point fluctuations in Figs 3 , 4 , 5 do support these stated levels of sampling error. Nevertheless, the general agreement of our results with those from other conventional approaches suggests that the errors in the present estimates do not seriously affect the conclusion that the eddy heat and salt transports are mainly due to individual eddy movements. The sampling errors will be reduced with more Argo profiles. Alternatively, the same methodology can be applied to a realistic, eddy-resolving global ocean model to reach more accurate estimates of eddy fluxes and their component due to eddy movement. Velocity geometry-based automated eddy detection scheme An eddy detection scheme based on velocity geometry has successfully been applied to data from a model [13] to SSHA-derived geostrophic velocity anomalies [10] and to SST-derived thermal wind velocity [11] . In a reference frame moving with the local mean velocity, an eddy is defined as a horizontal flow feature where the relative velocity vectors rotate around a centre. The velocity field associated with an eddy is characterized by a velocity minimum in the centre and by a tangential velocity increasing linearly with the distance from the centre and then deceasing after reaching a maximum value. Furthermore, because of the rotational structure of an eddy flow, the ( u , v ) components reverse in sign across the eddy centre. Eddy detection depends on sufficient conformity with these flow criteria. This method also provides an eddy-tracking scheme based on time continuity of an individual eddy detection. Estimation of heat and salt transports by eddy movement The following procedure is applied in the present study to estimate the heat and salt transport by eddy movement: (1) using the automated eddy detection scheme [13] , a global eddy data set is determined from altimetric SSHA; (2) mean vertical profiles of sea water T/S are estimated in 5° × 5° bins using all available Argo profiles; (3) the T/S vertical profile anomalies ( T ′, S ′) are calculated for each eddy that contains Argo profiles; (4) the heat and salt transports by the movement of each eddy containing Argo profiles, ( Q eh , Q es ), are calculated from (1), and then the average heat and salt transports per eddy and the s.d. are calculated in 5° × 5° bins; (5) from altimetric SSHA detections, the total eddy population in the bins is calculated, along with the total heat and salt (freshwater) transports due to eddy movement (2); and (6) with the s.d. in each bin from step (4), the uncertainty for each zonal band is calculated using the following formula: where Δ b is the uncertainty of the heat (freshwater) transport in a zonal band (the subscript b denotes the b th band of all zonal bands); σ i is the s.d. of the transport in one bin (the subscript i denotes the i th of all bins in Band b ; n b is the number of bins in Band b ; δ is an in situ measurement error associated with the co-located Argo profiles and satellite data. However, quantifying the measurement errors is beyond the scope of the study, and therefore δ is not included in the calculation for Figs 4 and 5 . How to cite this article: Dong, C. et al. Global heat and salt transports by eddy movement. Nat. Commun. 5:3294 doi: 10.1038/ncomms4294 (2013).